Metformin elicits anticancer effects through the sequential modulation of DICER and c-MYC Diabetic patients treated with metformin have a reduced incidence of cancer and cancer-related mortality. Here we show that metformin affects engraftment and growth of breast cancer tumours in mice. This correlates with the induction of metabolic changes compatible with clear anticancer effects. We demonstrate that microRNA modulation underlies the anticancer metabolic actions of metformin. In fact, metformin induces DICER expression and its effects are severely impaired in DICER knocked down cells. Conversely, ectopic expression of DICER recapitulates the effects of metformin in vivo and in vitro . The microRNAs upregulated by metformin belong mainly to energy metabolism pathways. Among the messenger RNAs downregulated by metformin, we found c-MYC, IRS-2 and HIF1alpha. Downregulation of c-MYC requires AMP-activated protein kinase-signalling and mir33a upregulation by metformin. Ectopic expression of c-MYC attenuates the anticancer metabolic effects of metformin. We suggest that DICER modulation, mir33a upregulation and c-MYC targeting have an important role in the anticancer metabolic effects of metformin. Altered metabolism is a key feature of cancer cells. It drives the cells towards a pro-proliferative anabolic phase rather than efficient ATP production. A distinct trait of the cancer metabolism is the unscheduled activation of glycolytic enzymes in normoxic conditions, indicated by increased cellular glucose uptake, hyper-glycolysis and lactate [1] , [2] , [3] . This represents a mechanism of neoplastic progression. Indeed, known oncogenes alter cell metabolism through modulation of key glycolytic enzymes [4] , [5] , [6] , [7] , [8] , [9] . Metformin (1,1–dimethylbiguanide hydrochloride) is a widely used antidiabetic agent that decreases insulin resistance and lowers blood glucose levels through the inhibition of liver glucose production and an increased glucose uptake in muscles [10] , [11] . Multiple epidemiological studies show that diabetic patients treated with metformin have reduced incidence of cancer and reduced cancer mortality [12] . In addition, metformin affects the progression and relapse of breast, prostate and lung cancer mouse xenografts, when combined with suboptimal doses of standard chemotherapeutic agents [13] , [14] , [15] , [16] . Metformin activates the AMP-activated protein kinase (AMPK) [17] , [18] , a major sensor of the energetic status of the cell [19] . Activation of AMPK inhibits mammalian target of rapamycin (mTOR) signalling [20] and stimulates the p53/p21 axis [21] potentially affecting p53 downstream targets [22] . Hence, metformin combines both metabolic and anticancer properties. Additionally, the anticancer activity of metformin on tumour xenografts highly differing in their tissue of origin, oncogene expression and p53 status [23] , [24] suggests the existence of a broader mechanism of action for this drug. MicroRNAs are short, stable, noncoding RNAs that target the mRNA of coding genes for degradation, thus effectively reducing the levels of the gene products. MicroRNA modulation represents an effective strategy through which external stimuli can rapidly alter the cell and tissue homeostasis, by targeting multiple genes at the same time. The RNAse III DICER has a role in processing double-stranded RNA to short interfering RNA (siRNA) and in the assembly of the siRNA into the machinery that targets the mRNAs for degradation [25] . In fact, the expression of DICER directly influences the biosynthesis of all microRNAs, thereby severely affecting gene expression patterns [26] . Interestingly, downregulation of the DICER levels was shown to represent an intrinsically oncogenic event, by enhancing epithelial to mesenchymal transition and metastatic dissemination of breast cancer cells [27] . Furthermore, low expression of DICER predicted poor survival of breast, lung and ovarian cancer patients [28] , [29] . Given the potential ability of metformin to broadly affect multiple pathways, we hypothesized that microRNA modulation could be part of its mechanism of action. By using xenograft transplantation experiments, hydrogen-( 1 H) nuclear magnetic resonance ( 1 H-NMR)-based metabolic analysis and microRNA profiling, we demonstrated that microRNA modulation underlies the anticancer metabolic actions of metformin. Metformin modulated microRNA by transcriptionally activating the promoter of DICER. Metformin-modulated microRNAs were predicted to impinge mainly on the energy metabolism and insulin signalling pathways. In addition, we show that metformin affects the mRNA levels of c-MYC, IRS-2 and HIF1alpha as well. The sequential modulation of DICER, microRNA-33a and of c-MYC levels may partially explain the anticancer metabolic effects of metformin. Metformin inhibits tumour engraftment and growth We performed experiments aimed at evaluating the effect of metformin on breast cancer xenografts. For this, we used a basal-like, triple-negative breast cancer cell line (SUM159PT) [30] and evaluated the effects of metformin in three different experimental settings ( Fig. 1 ). First, we studied the frequency of tumour engraftment in metformin-pretreated mice. 1 week before cell transplantation, mice ( n =7) were treated intraperitoneally with either metformin (16 mg kg −1 ) or vehicle ( Fig. 1a ) and metformin treatment restarted 72 h after cell implantation up to the termination of the study (day 121). The tumour engraftment in mice pretreated with metformin was significantly reduced (6/7 and 2/7 engrafted tumours for vehicle- and metformin-treated mice, respectively, P <0.05; Fig. 1a ). A clear effect of metformin on the survival of tumour-bearing mice was observed as well ( Fig. 1b ). Second, to study the effect on tumour incidence, we evaluated the impact of metformin on tumour re-engraftment. In short, tumours collected from either treated or untreated mice (as from 1a,b) were enzymatically digested and re-transplanted into new untreated-recipient hosts ( n =7). This revealed that the engraftment rate of the tumours excised from metformin-treated donors was considerably reduced, as compared with that of the tumours derived from vehicle-treated donors (7/7 and 3/7 engrafted tumours for vehicle- and metformin-treated mice, respectively, P <0.05; Fig. 1c ). Third, we evaluated the effect of metformin (16 mg kg −1 , bi-weekly) in comparison to that of doxorubicin (4 mg kg −1 , weekly) on already established tumours (starting volume±0.2 cm 3 ) ( Fig. 1d ). This showed that metformin-treated mice had smaller tumours than vehicle-treated mice (0.85±0.09 cm 3 vs 2,33±0.24 cm 3 , at day 60 p.i., respectively) and that metformin-treatment affected tumour volume to a degree comparable to doxorubicin treatment (0.85±0.09 cm 3 vs 1.20±0.09 cm 3 at day 60 post cell injection, respectively). Finally, the proliferative index of tumours derived from metformin-treated mice was much lower than that of control mice ( Fig. 1e,f ). Interestingly, no toxicity was observed in mice treated with metformin ( Fig. 1b ). 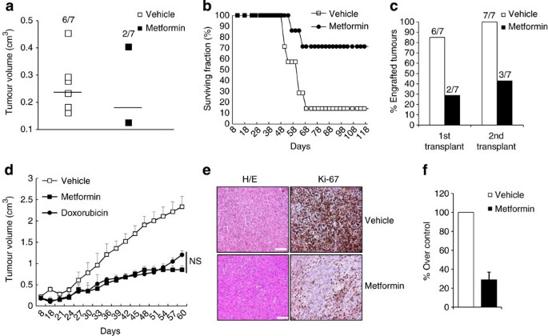Figure 1: Anticancer properties of metformin. (a) Tumour volume of CD1 mice treated with vehicle or metformin (16 mg kg−1, bi-weekly) before subcutaneous transplantation of SUM159PT cells (1×106cells per mouse,n=7). (b) Survival curve of the CD1 mice (n=7) as from the experiment in (a). Log-rank test used to compare survival curves (P<0.05). (c) Tumour re-engraftment assay. Briefly, tumours (n=2 per group) excised from the mice as from (a) (first transplant) were disaggregated and transplanted into untreated secondary recipient mice (second transplant,n=7). Histograms show the percentage of re-engrafted tumours in untreated recipients. (d) Tumour volume of mice (n=6) treated with doxorubicin (4 mg kg−1- for 4 *5dd cycles) or metformin (16 mg kg−1, biweekly) when the average starting tumour volume was 0.2 cm3. (e) Representative micrographs of the excised tumours at day 60 p.i. Scale bar, 100 μm. (f) Histograms show the percentage of positive cells from four tumours per group. Mean±s.d. values represent the average of three independent experiments Statistics:P<0.05 by Student'st-test. NS, not significant. Figure 1: Anticancer properties of metformin. ( a ) Tumour volume of CD1 mice treated with vehicle or metformin (16 mg kg −1 , bi-weekly) before subcutaneous transplantation of SUM159PT cells (1×10 6 cells per mouse, n =7). ( b ) Survival curve of the CD1 mice ( n =7) as from the experiment in ( a ). Log-rank test used to compare survival curves ( P <0.05). ( c ) Tumour re-engraftment assay. Briefly, tumours ( n =2 per group) excised from the mice as from ( a ) (first transplant) were disaggregated and transplanted into untreated secondary recipient mice (second transplant, n =7). Histograms show the percentage of re-engrafted tumours in untreated recipients. ( d ) Tumour volume of mice ( n =6) treated with doxorubicin (4 mg kg −1 - for 4 *5dd cycles) or metformin (16 mg kg −1 , biweekly) when the average starting tumour volume was 0.2 cm 3 . ( e ) Representative micrographs of the excised tumours at day 60 p.i. Scale bar, 100 μm. ( f ) Histograms show the percentage of positive cells from four tumours per group. Mean±s.d. values represent the average of three independent experiments Statistics: P <0.05 by Student's t -test. NS, not significant. Full size image Metformin has anticancer metabolic effects We then used 1 H-NMR spectroscopy [31] , [32] , [33] to characterize the metabolic effects of metformin. In short, we collected the NMR spectra of drug- and vehicle-treated samples from tumour tissue extracts ( Fig. 2a–c ) and the data were organized according to a principal component analysis (PCA) model, an unsupervised method allowing orthogonal decomposition of variance associated with the analysed metabolites [34] . This revealed that the metabolic effects of metformin were different from those exerted by doxorubicin treatment ( Fig. 2a ; Supplementary Table S1 ). More in detail, the orthogonal projections to latent structures-discriminant analysis (OPLS-DA) [35] (that excludes from the analysis the background metabolic effects not due to metformin) revealed that vehicle- and metformin-treated tumour samples were significantly different on the first component ( t 0 ), which describes the funnelling of glucose, glutamate and pyruvate to sustain energy production ( Fig. 2b ). Therefore, the metformin-treated tumours bore significant differences in the way glucose is used and how carbon (from glucose) is funnelled through the central carbon metabolism (Glycolysis, the pentose phosphate pathway and the TCA cycle). 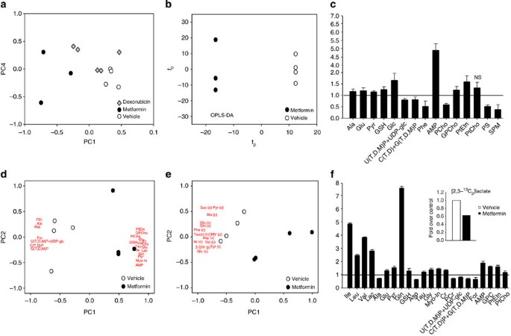Figure 2: Metabolic effects of metformin. (a–c)1H-NMR determination of the metabolites of the excised tumours from vehicle-, doxorubicin- or metformin-treated mice. NMR data were organized according to a principal component analysis (PCA) model. Metabolite clustering identifies pathways (KEGG) and the association of metabolites with vehicle- or metformin-treated samples (empty symbols vs filled symbols, respectively) indicates pathway engagement. In (b), an OPLS-DA analysis was used to minimize the effect of the background signal in the excised tumours. (c) Histograms indicate the relative levels of the main metabolites considered in the score/loading plots in (b) (d–f)1H-NMR determination of the metabolites fromin vitrocultured SUM159PT cells. (d) PCA score/loading plots for the intracellular metabolites of vehicle and metformin-treated cells. (e) PCA-score/loading plots for the extracellular metabolites of vehicle and metformin-treated cells. (f) Histograms showing the relative levels of the main metabolites considered in (d). (f) inset: relative levels of glucose-derived lactate from SUM159PT cells labelled with [1,2-13C2]-glucose. Data represent mean±s.d. values of at least three independent experiments. Statistics:P<0.05. NS, not significant. Ala, alanine; Glu, glutamate; Pyr, pyruvate; GSH, glutathione, Glc, glucose; Phe, phenylalanine; U(T,D,M)P+UDP-glc, uridine triphosphate, diphosphate and monophosphate + uridine diphosphate glucose; C(T,D)+G(T,D,M)P, cytidine triphosphate and diphosphate + guanosine triphosphate, diphosphate and monophosphate; AMP, adenosine monophosphate; PtCho, phosphatidylcholine; PtEN, phosphatidyl-ethanolamine; PS, serine phospholipids; SPH, sphingomyelin. Specifically, our analysis showed a reduced utilization of the pentose-phosphate-pathway for the nucleotide synthesis in metformin-treated tumours ( Fig 2c ). We observed a perturbation of phospholipid and sphingolipid metabolism: with a significantly higher glycerophosphocholine to phosphocholine (GPC to PC) ratio in metformin-treated tumours (1.10±0.06 and 0.76±0.17 for metformin and vehicle-treated mice, respectively, P <0.02; Fig. 2c ). Interestingly, a higher GPC to PC ratio is a feature of non-tumour cells [36] , [37] . Overall, the in vivo analysis suggested a shift from a mainly anabolic to a more catabolic utilization of glucose-derived carbon in metformin-treated cells. We provided a more detailed characterization of the metabolic fluxes modulated by metformin by analysing the changes of intracellular and extracellular metabolites in in vitro cultured SUM159PT cells ( Fig. 2d–f ). Cells were exposed to concentrations of metformin (0.5 mM) that did not cause any measurable cytotoxic effect, while promoting activation of the AMPK pathway ( Supplementary Fig. S1 ). A statistically significant separation between the two groups of samples was observed on the PC1 ( P <0.001; Fig. 2d ). Analysis of the loading plots on the PC1 revealed that, as compared with vehicle-treated cells, metformin-treated cells showed higher levels of branched-chain amino acids, lactate, glutamine, glutamate, pyruvate, glycine, glutathione, taurine, myo-inositol, creatine, glycerophosphocholine, phosphatidyl-choline, phosphatidyl-ethanolamine and AMP (positive correlation with PC1) as well as lower levels of alanine, aspartate, formate, phosphocreatine and nucleotides (negative correlation with PC1, Fig. 2d, f ). High levels of AMP in the metformin-treated samples indicated a decreased ATP/AMP ratio, which may highlight AMPK activation ( Fig. 2f ). In line with this, we observed increased levels of creatine and reduced levels of phosphocreatine in the treated cells, consistent with a decreased storage of intracellular ATP ( Fig. 2f ). The in vitro analysis indicated a decreased ATP storage and a reduced de novo nucleotide synthesis. We then analysed the NMR spectra of conditioned media from vehicle- and metformin-treated SUM159PT cells ( Fig. 2e ). The analysis of the metabolite loadings revealed that metformin treatment induced higher consumption of branched-chain amino acids, glutamine, glutamate, succinate, aspartate, glucose, tyrosine and phenylalanine as well as a lower production of ketoacids (2-OMV and 2-OIV) ( Fig. 2e ). As 2-OMV and 2-OIV are catabolic intermediates of the branched-chain amino acids, this indicated that the treated cells convert preferentially isoleucine and valine to succinyl-CoA. This suggested that metformin-treated cells use amino acids for energy production, instead of macromolecule biosynthesis. In summary, the in vitro data suggested a reversion from anabolic to catabolic metabolism, thus recapitulating what previously observed in vivo. Interestingly, the combined analysis of the extracellular and intracellular metabolites showed that metformin-treated cells took up more glucose and produced more lactate. However, a lower flux of metabolites through the glycolysis in metformin-treated samples was observed ( Fig. 2d–e ). This was confirmed by the NMR analysis with [1,2- 13 C 2 ]-glucose, showing that the levels of glucose-derived lactate were lower in metformin-treated samples as compared with vehicle-treated cells ( Fig. 2f , inset). Therefore, in the treated cells, glucose was used mainly for catabolic purposes rather than for nucleotide biosynthesis. Interestingly, metformin treatment affected similarly the metabolic profile of two unrelated breast cancer cell lines (MCF-7 and BT-474), with the strongest effect observed for MCF7 cells on the PC2. PC2 (0.06 for SUM159PT, 0.45 for MCF-7, and 0.27 for BT-474- Supplementary Fig. S2a ; Supplementary Table S2 ). We observed no significant effect of the drug on the metabolic activity of MCF10A cells (untransformed, dysplastic breast cells) [38] ( Supplementary Fig. S2a ; Supplementary Table S2 ). This correlated with the absence of toxic effects observed in metformin-treated mice ( Fig. 1b ). Figure 2: Metabolic effects of metformin. ( a–c ) 1 H-NMR determination of the metabolites of the excised tumours from vehicle-, doxorubicin- or metformin-treated mice. NMR data were organized according to a principal component analysis (PCA) model. Metabolite clustering identifies pathways (KEGG) and the association of metabolites with vehicle- or metformin-treated samples (empty symbols vs filled symbols, respectively) indicates pathway engagement. In ( b ), an OPLS-DA analysis was used to minimize the effect of the background signal in the excised tumours. ( c ) Histograms indicate the relative levels of the main metabolites considered in the score/loading plots in ( b ) ( d–f ) 1 H-NMR determination of the metabolites from in vitro cultured SUM159PT cells. ( d ) PCA score/loading plots for the intracellular metabolites of vehicle and metformin-treated cells. ( e ) PCA-score/loading plots for the extracellular metabolites of vehicle and metformin-treated cells. ( f ) Histograms showing the relative levels of the main metabolites considered in ( d ). ( f ) inset: relative levels of glucose-derived lactate from SUM159PT cells labelled with [1,2- 13 C 2 ]-glucose. Data represent mean±s.d. values of at least three independent experiments. Statistics: P <0.05. NS, not significant. Ala, alanine; Glu, glutamate; Pyr, pyruvate; GSH, glutathione, Glc, glucose; Phe, phenylalanine; U(T,D,M)P+UDP-glc, uridine triphosphate, diphosphate and monophosphate + uridine diphosphate glucose; C(T,D)+G(T,D,M)P, cytidine triphosphate and diphosphate + guanosine triphosphate, diphosphate and monophosphate; AMP, adenosine monophosphate; PtCho, phosphatidylcholine; PtEN, phosphatidyl-ethanolamine; PS, serine phospholipids; SPH, sphingomyelin. Full size image Metformin modulates microRNAs To investigate which mechanisms could underlie the observed effects of metformin, we studied the microRNA expression of vehicle- and metformin-treated breast cancer cells, by using the same experimental conditions used for the metabolic profiling ( Fig. 2d-f ). Metformin treatment affected microRNA expression of all the breast cancer cell lines tested, with no statistically significant modulation only in the dysplastic MCF10A cells (ANOVA analysis, P <0.05; Supplementary Fig. S2b ). A more detailed analysis of the SUM159PT cells treated with metformin revealed a change of the overall microRNA levels ( Fig. 3a ; Supplementary data 1 ) that was attenuated in those cells stably infected with DICER-targeting short hairpin RNAs (shRNAs)(referred as DICER k/d cells in Fig. 3b ). 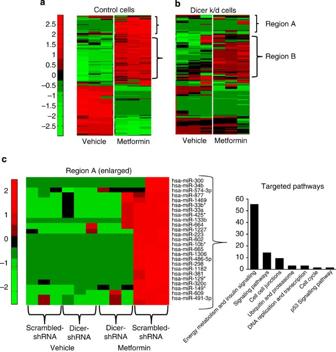Figure 3: Metformin modulates microRNAs. (a,b) Heat maps depicting microRNA levels of bulk SUM159PT cells stably expressing either a control (scrambled)-shRNA (a) or a DICER-targeting shRNA (b) and treated with vehicle or metformin for 24 h. (c) Enlarged image of the region 'A' with indication of the single microRNAs analysed.In silicoprediction of the pathways affected by metformin-regulated microRNAs (http://diana.cslab.ece.ntua.gr). Manual annotation of the breast-specific pathways. As expected, DICER depletion did not seem to affect microRNAs, whose levels were low at steady state ( Fig 3b ). Among the microRNAs upregulated by metformin in SUM159PT cells, two different groups (regions A and B) could be observed, based on their apparent sensitivity to DICER depletion ( Fig. 3a,b ). We focussed on the microRNAs upregulated by metformin in the region A of the clustergram, which showed the highest level of sensitivity to DICER depletion ( Fig. 3b ). In silico prediction analysis revealed that the microRNAs in the selected region mostly targeted genes involved in metabolism and insulin signalling ( Fig. 3c ), thus establishing a link between the microRNA modulation and the metabolic action of the drug. Figure 3: Metformin modulates microRNAs. ( a,b ) Heat maps depicting microRNA levels of bulk SUM159PT cells stably expressing either a control (scrambled)-shRNA ( a ) or a DICER-targeting shRNA ( b ) and treated with vehicle or metformin for 24 h. ( c ) Enlarged image of the region 'A' with indication of the single microRNAs analysed. In silico prediction of the pathways affected by metformin-regulated microRNAs ( http://diana.cslab.ece.ntua.gr ). Manual annotation of the breast-specific pathways. Full size image Metformin modulates the levels of DICER To understand how metformin could modulate the levels of the intracellular microRNAs, we evaluated the effect of metformin on the RNASE III endonuclease DICER, one of the key enzymes of microRNA biogenesis [26] . We found that treatment of SUM159PT cells with metformin for 24 h led to a significant increase in DICER protein levels ( Fig. 4a ) that correlated with increased mRNA levels of DICER ( Fig. 4b ). Two other known AMPK activators (phenformin and AICAR) affected DICER levels as well ( Fig. 4c ). A computer-assisted analysis of the DICER promoter (promoter 1) revealed the presence of multiple E2F DNA-binding sites within 1 kb from the transcription start site ( Fig. 4d ). We hypothesized that metformin could influence the activity of the E2F transcription factors on the DICER promoter. To this end, we performed chromatin immunoprecipitation experiments aimed at evaluating promoter occupancy by E2F transcription factors in the treated cells. This showed that metformin treatment triggered an increased binding of the transcriptional activator E2F3 while promoting a decrease of the transcriptional repressor E2F5 at the DICER promoter ( Fig. 4d–e ). Additionally, the presence of the hyper-acetylated histone H4, of the histone acetyl-transferase p300 and of the elongating form of Pol-II (pol-II phospho-CTDser2) was increased at the E2F binding sites in the treated cells, indicating transcriptional activation of the promoter by metformin ( Fig. 4f ). To confirm the role of the E2Fs in mediating the increase of DICER in metformin-treated cells, we depleted by siRNA the E2F1/E2F3 in 293 cells and this affected the induction of DICER mRNA by metformin ( Fig. 4g ). Conversely, the overexpression of E2F1 and E2F3 triggered an induction of DICER mRNA compatible with that observed on metformin treatment ( Fig. 4h ). 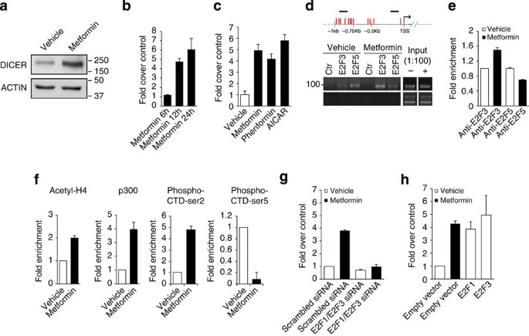Figure 4: Metformin modulates the levels of DICER. (a) Western blotting with anti-DICER antibodies of whole cell lysates from SUM159PT cells treated with vehicle or metformin for 24 h. Actin staining was used as a loading control. (b, c). qPCR. mRNA levels of DICER from SUM159PT cells treated with metformin at the indicated times (b) or treated with AMPK activators for 12 h (c). (d) Predicted E2F binding sites in the DICER promoter. Horizontal bars indicate the regions amplified in the CHIP experiment. Representative image of a CHIP assay with the indicated antibodies from SUM159PT cells treated as above. (e) Histograms showing densitometric evaluation of two independent CHIP experiments. (f) qPCR: amplification of E2F binding sites from CHIP assays with the indicated antibodies from vehicle and metformin-treated cells. (g) qPCR: mRNA levels of DICER from 293T cells transfected with either scrambled-siRNA and E2F1/E2F3 targeting siRNAs and treated as indicated. (h) qPCR. mRNA levels of DICER from 293T cells transfected with either empty vector (and treated as indicated) or with E2F1- and E2F3-expressing vectors. Mean±s.d. values represent the average of three independent experiments. Statistics:P<0.05 by Student'st-test. Figure 4: Metformin modulates the levels of DICER. ( a ) Western blotting with anti-DICER antibodies of whole cell lysates from SUM159PT cells treated with vehicle or metformin for 24 h. Actin staining was used as a loading control. ( b, c ). qPCR. mRNA levels of DICER from SUM159PT cells treated with metformin at the indicated times ( b ) or treated with AMPK activators for 12 h ( c ). ( d ) Predicted E2F binding sites in the DICER promoter. Horizontal bars indicate the regions amplified in the CHIP experiment. Representative image of a CHIP assay with the indicated antibodies from SUM159PT cells treated as above. ( e ) Histograms showing densitometric evaluation of two independent CHIP experiments. ( f ) qPCR: amplification of E2F binding sites from CHIP assays with the indicated antibodies from vehicle and metformin-treated cells. ( g ) qPCR: mRNA levels of DICER from 293T cells transfected with either scrambled-siRNA and E2F1/E2F3 targeting siRNAs and treated as indicated. ( h ) qPCR. mRNA levels of DICER from 293T cells transfected with either empty vector (and treated as indicated) or with E2F1- and E2F3-expressing vectors. Mean±s.d. values represent the average of three independent experiments. Statistics: P <0.05 by Student's t -test. Full size image DICER is required for the anticancer action of metformin To study the functional relevance of DICER modulation for the anticancer effects of metformin, we evaluated the effect of the drug on the tumorigenic properties of control (scrambled-shRNA)- and DICER k/d SUM159PT cells ( Fig. 5a ). 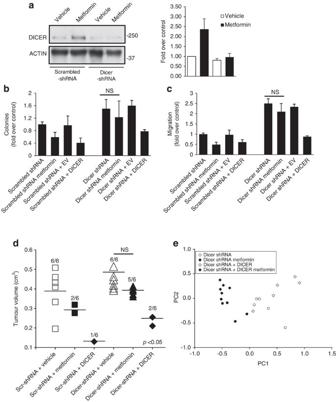Figure 5: DICER modulation mediates the anticancer metabolic effects of metformin. (a) Western blotting with anti-DICER antibodies of whole cell lysates from the indicated SUM159PT cells treated with vehicle or metformin for 24 h. Actin staining was used as a loading control. (b,c) Histograms showing the average results of three independent clonogenic (b) or wound healing (c) assays from the indicated SUM159PT cells treated as indicated. Statistics:P<0.05 by Student'st-test. NS, not significant (d) Tumour volumes (day 55p.i.) of CD1 mice treated with vehicle- or metformin (16 mg kg−1, bi-weekly) before subcutaneous transplantation of the indicated SUM159PT cell lines. Tumours with volume >0.1 cm3were considered as engrafted. The engrafted to injected mice ratio is reported for each group. The horizontal bars indicate the mean volume of the engrafted tumours. Statistics:P<0.05 by Student'st-test. NS, not significant. (e)1H-NMR footprinting and PCA analysis of the extracellular metabolites from DICER k/d SUM159PT cells transfected as indicated and treated with metformin. This revealed that metformin treatment affected both colony-forming ability and wound-healing closure of control cells, thus pairing the observed effect on the engraftment of newly formed tumours and that these effects were strongly attenuated in DICER k/d cells ( Fig 5b-c, Supplementary Fig. S4a,b ). Notably, the ectopic expression of an RNAi-resistant DICER mRNA affected the clonogenicity and the migration of SUM159PT cells in a way similar to metformin treatment ( Fig. 5b–c ). Next, we compared the effect of metformin and that of the ectopic expression of the RNAi-resistant DICER on the engraftment of control- and DICER k/d cells. The in vivo study revealed that metformin affected tumour engraftment in control cells and was unable to do so in DICER k/d cells (2/6 vs 5/6 engrafted tumours/injected mice in metformin-treated control and DICER k/d cells, respectively; Fig. 5d ). Additionally, the overexpression of the RNAi-stable DICER in both control and DICER k/d cells affected the tumour engraftment in a way comparable to the metformin treatment ( Fig. 5d ). Finally, we evaluated whether the ectopic expression of RNAi-stable DICER could rescue the effect of metformin on the DICER k/d cells. The overexpression of the RNAi-resistant DICER in DICER k/d cells affected the metabolic profile of the cells with major changes on the PC1 ( Fig. 5e ; Supplementary Table S3 ). Moreover, metformin treatment triggered stronger metabolic changes on the PC1 in the DICER k/d cells transfected with the RNAi-resistant DICER, as compared with those transfected with the empty-vector ( P =0.001 vs 0.01, respectively ( Fig. 5e ; Supplementary Table S3) ). Thus, both ectopic expression of DICER and metformin treatment perturbed similar metabolic components and showed synergistic effects on the PC1 ( Fig. 5e ; Supplementary Table S3 ). This correlated with the observation that many metformin-modulated microRNAs target energy metabolism pathways ( Fig. 3c ). In summary, ectopic expression of DICER mimicked, to a considerable extent, the effect of metformin in terms of metabolic modulation, tumour engraftment, colony-forming ability and wound-healing inhibition. Figure 5: DICER modulation mediates the anticancer metabolic effects of metformin. ( a ) Western blotting with anti-DICER antibodies of whole cell lysates from the indicated SUM159PT cells treated with vehicle or metformin for 24 h. Actin staining was used as a loading control. ( b,c ) Histograms showing the average results of three independent clonogenic ( b ) or wound healing ( c ) assays from the indicated SUM159PT cells treated as indicated. Statistics: P <0.05 by Student's t -test. NS, not significant ( d ) Tumour volumes (day 55p.i.) of CD1 mice treated with vehicle- or metformin (16 mg kg −1 , bi-weekly) before subcutaneous transplantation of the indicated SUM159PT cell lines. Tumours with volume >0.1 cm 3 were considered as engrafted. The engrafted to injected mice ratio is reported for each group. The horizontal bars indicate the mean volume of the engrafted tumours. Statistics: P <0.05 by Student's t -test. NS, not significant. ( e ) 1 H-NMR footprinting and PCA analysis of the extracellular metabolites from DICER k/d SUM159PT cells transfected as indicated and treated with metformin. Full size image Metformin modulates c-MYC levels via mir-33a Among the metformin-regulated microRNAs, we focussed on the microRNA-33a owing to its robust modulation by metformin (~4-folds-log2- over vehicle-treated cells, Supplementary data 1 , bold), its predicted binding to the c-MYC-UTR region (position 80–86 in the inset of Fig. 6a ), and its involvement into the modulation of IRS2 levels [39] . Quantitative PCR (qPCR) revealed that metformin and two other AMPK activators (phenformin and AICAR) altered the microRNA-33a levels and this was abolished in DICER k/d cells ( Fig. 6a ). Upregulation of mir-33a by metformin paired with a downregulation of the 3′UTR activity of the c-MYC mRNA, which was specifically antagonized by a mir33a antagonist ( Fig. 6b ). Consequently, metformin significantly downregulated the endogenous c-MYC mRNA and protein levels in a DICER-dependent way ( Fig. 6c-d, upper panel). 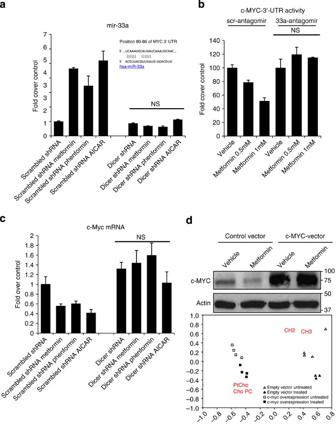Figure 6: Metformin modulates mir33a and c-MYC levels. (a) qPCR: Mir33a levels from the indicated SUM159PT-derived cell lines treated as indicated. Inset shows the mir-33a binding region. (b) Metformin modulates c-MYC-3′UTR activity. 293T cells co-transfected with the c-MYC 3-UTR luciferase reporter and either a scrambled- or a specific mir33a-antagonist. Histograms show the normalized luciferase values from three independent experiments. (c) qPCR. mRNA levels of c-MYC from the indicated SUM159PT-derived cell lines treated as indicated. Mean±s.d. values represent the average of three independent experiments. Statistics:P<0.05 by Student'st-test. NS: not significant (d) Overexpression of c-MYC attenuates metformin-induced metabolic effects. Upper panel. WB with anti-c-MYC antibodies of whole cell lysates from SUM159PT cells were stably transfected as indicated. WB anti-actin as a loading control. Lower panel.1H-NMR/PCA analysis of the cells as from the upper panel. Figure 6: Metformin modulates mir33a and c-MYC levels. ( a ) qPCR: Mir33a levels from the indicated SUM159PT-derived cell lines treated as indicated. Inset shows the mir-33a binding region. ( b ) Metformin modulates c-MYC-3′UTR activity. 293T cells co-transfected with the c-MYC 3-UTR luciferase reporter and either a scrambled- or a specific mir33a-antagonist. Histograms show the normalized luciferase values from three independent experiments. ( c ) qPCR. mRNA levels of c-MYC from the indicated SUM159PT-derived cell lines treated as indicated. Mean±s.d. values represent the average of three independent experiments. Statistics: P <0.05 by Student's t -test. NS: not significant ( d ) Overexpression of c-MYC attenuates metformin-induced metabolic effects. Upper panel. WB with anti-c-MYC antibodies of whole cell lysates from SUM159PT cells were stably transfected as indicated. WB anti-actin as a loading control. Lower panel. 1 H-NMR/PCA analysis of the cells as from the upper panel. Full size image Modulation of c-MYC mediates the metabolic effect of metformin Finally, we tested whether the ectopic expression of c-MYC could counteract the metabolic effects of metformin. To this end, we stably transfected SUM159PT cells with either empty- or c-MYC-expressing vectors and treated them with vehicle or metformin ( Fig. 6d ). The analysis of the extracellular metabolites revealed that, in c-MYC-overexpressing cells, the effect of metformin was significantly attenuated on the PC2. In fact, the average distance from the center of metformin-treated control- and c-MYC overexpressing samples was 0.60 and 0.43, respectively, on the PC2 axis (arbitrary units- P <0.01); Supplementary Table S4 ). Altogether, these data suggest that modulation of the mRNA and protein levels of c-MYC is AMPK- and DICER-dependent and relevant for the metabolic anticancer effect of metformin. According to a recently published work involving mir33a in the regulation of IRS2 mRNA [37] , we found that metformin treatment affected the mRNA and protein levels of IRS2 as well ( Fig. 7 ). Additionally, as c-MYC is shown to synergize with HIF1 alpha to promote aerobic glycolysis and glutaminolysis [40] , [41] , we tested whether metformin could alter the levels of HIF1alpha. This showed that metformin affected significantly the mRNA and protein levels of HIF1alpha in hypoxic SUM159PT cells ( Fig. 7 ). 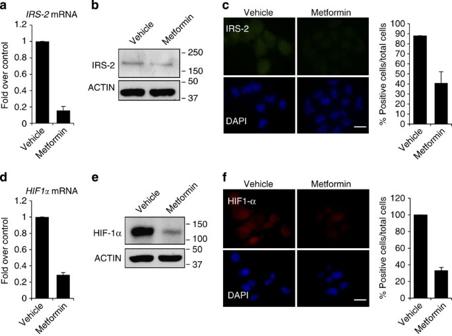Figure 7: Metformin modulates the levels of IRS-2 and HIF1alpha. (a) qPCR. mRNA levels of IRS2 from the indicated SUM159PT cell lines treated with metformin for 24 h. (b) Western blotting with anti-IRS2 antibodies of WCL from the indicated SUM159PT cell lines treated with vehicle or metformin. Actin staining was used as a loading control. (c) Indirect Immunofluorescence of SUM159PT cell treated as indicated and stained with anti-IRS2 antibody. Scale bar, 20 μm. (d) qPCR. mRNA levels of HIF1α from the indicated SUM159PT cell lines treated with metformin for 24 h. (e) Western blotting with anti-HIF1alpha antibodies of WCL from the SUM159PT cell lines treated with vehicle or metformin. Actin staining as a loading control. (f) Indirect immunofluorescence of SUM159PT cells treated as indicated and stained with anti-HIF1alpha antibodies. Scale bar, 20 μm. In (c) and (f), histograms showing the percentage of positive cells per total cells from triplicate experiments. In (d–f), cells were previously grown for 16 h in hypoxic conditions as indicated in methods. Statistics:P<0.05 by Student'st-test. Figure 7: Metformin modulates the levels of IRS-2 and HIF1alpha. ( a ) qPCR. mRNA levels of IRS2 from the indicated SUM159PT cell lines treated with metformin for 24 h. ( b ) Western blotting with anti-IRS2 antibodies of WCL from the indicated SUM159PT cell lines treated with vehicle or metformin. Actin staining was used as a loading control. ( c ) Indirect Immunofluorescence of SUM159PT cell treated as indicated and stained with anti-IRS2 antibody. Scale bar, 20 μm. ( d ) qPCR. mRNA levels of HIF1α from the indicated SUM159PT cell lines treated with metformin for 24 h. ( e ) Western blotting with anti-HIF1alpha antibodies of WCL from the SUM159PT cell lines treated with vehicle or metformin. Actin staining as a loading control. ( f ) Indirect immunofluorescence of SUM159PT cells treated as indicated and stained with anti-HIF1alpha antibodies. Scale bar, 20 μm. In ( c ) and ( f ), histograms showing the percentage of positive cells per total cells from triplicate experiments. In ( d–f ), cells were previously grown for 16 h in hypoxic conditions as indicated in methods. Statistics: P <0.05 by Student's t -test. Full size image Over the last 30 years, metformin has been widely used as an antidiabetic agent owing to its relatively mild adverse effects and its effective mechanism of action on insulin and glucose levels. Recent studies have shown an effect of metformin on tumour-repopulating cell subpopulations [16] , and ample epidemiological data documented a reduced cancer incidence and cancer mortality in metformin-treated diabetic patients [11] . The molecular relationships between the metabolic and anticancer actions of metformin are still poorly defined. In this work, we aimed at investigating a mechanistic link between the metabolic action of metformin and its anticancer effects. We carried out xenograft transplantation studies, and we found that metformin strongly inhibited both the engraftment and re-engraftment of SUM159PT-driven tumours and reduced the growth of already established tumours ( Fig. 1 ). Coupling of 1 H-NMR metabolic-foot-printing to the xenograft experiments revealed that metformin elicited a number of metabolic changes compatible with a clear anticancer effect ( Fig. 2 ). On the whole, this consisted of a reversion from the anabolic to the catabolic utilization of glucose, with a significantly reduced utilization of glucose for anabolic purposes (for example, nucleotide biosynthesis). In fact, pro-anabolic utilization of carbon-derived glucose is a feature of cancer tissues, required to sustain the increased requirement for macromolecule biosynthesis [42] . We set up suitable in vitro conditions (for multiple breast cancer cell lines) that strictly recapitulated the metabolic changes induced by metformin in the xenografted tumours ( Supplementary Fig. S2a ). This allowed us to identify microRNA modulation as an important feature of metformin treatment in three breast cancer cell lines differing for histological phenotype, p53 status and HER2 expression (MCF-7, BT474 and SUM159PT cells) ( Supplementary Fig. 2b ). Metformin was found ineffective in inducing statistically significant changes in both the metabolic profile and microRNA expression of dysplastic, untransformed MCF10A cells ( Supplementary Fig. 2a,b ). This recalls the absence of any toxic effect we observed in the treated mice and pairs with the observation that all the experiments were performed by using non-cytotoxic, clinically relevant concentrations of the drug ( Supplementary Fig. S1 ). Metformin surprisingly increases the dicer mRNA and protein levels and this is required for its anticancer effects in vivo and in vitro ( Figs 4 and 5 ; Supplementary Figs S3 and S4 ). Cancer cells often exhibit microRNA downregulation when compared with their normal counterparts. This may be mimicked by the shRNA- or microRNA-mediated knockdown of the dicer protein and correlates with the acquisition of tumorigenic properties [27] . Therefore, upregulation of the DICER levels by metformin may represent per se an important tumour-suppressor mechanism. The overexpression of DICER recapitulated largely, but not completely, the effects of the metformin treatment ( Fig. 5 ). This suggests that other dicer-independent mechanisms may be involved in the action of the drug and it may explain the paradoxical downregulation of several microRNAs even in the presence of increased levels of dicer in metformin-treated cells ( Fig. 3b ). Metformin affects the levels of c-MYC and this is mediated by the mir33a ( Fig. 8 ). c-MYC is a master regulator of cancer cell metabolism because of its effect on glycolytic and glutaminolytic anabolic pathways in cancer cells from various tissues [4] , [5] . Overexpression of c-MYC renders metformin-treated cells refractory to the metabolic effect of the drug, suggesting the functional relevance of c-MYC modulation for the effects of metformin ( Fig. 6 ). Metformin treatment affected the levels of HIF1alpha and IRS-2 as well ( Fig. 7 ). IRS-2 downregulation may be relevant for the interference of metformin with the insulin signalling and with cancer cell migration [43] , and can be mediated by the mir-33a [43] . Additionally, HIF1alpha is known to sustain aerobic glycolysis in metastatic cancer cells [8] , [41] and to cooperate with c-MYC [40] . All this unravels metformin's potential in tackling cancer cell metabolism by interfering with cooperative mechanisms ( Fig. 8 ). Given that altered metabolism is one of the most important characteristics of cancer, we believe this study suggests that a broader use of metabolic modulators such as metformin could have a major impact on the treatment of human tumours. 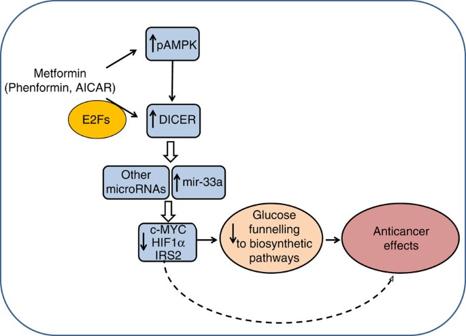Figure 8: Schematic model of the proposed mechanisms for the anticancer metabolic action of metformin. Solid lines indicate the proposed mechanisms as supported by the data presented. Dashed lines indicate additional mechanisms of action either already known or not investigated in the present manuscript. Figure 8: Schematic model of the proposed mechanisms for the anticancer metabolic action of metformin. Solid lines indicate the proposed mechanisms as supported by the data presented. Dashed lines indicate additional mechanisms of action either already known or not investigated in the present manuscript. Full size image Reagents Metformin (1,1-Dimethylbiguanide-hydrochloride) AICAR (5-Aminoimidazole-4-carboxamide-1-β-D-ribofuranoside), Phenformin (Phenethylbiguanide) and Doxorubicin-hydrochloride were purchased from Sigma-Aldrich. Cell culture conditions MCF-7 and BT-474 breast cancer cell lines were grown in DMEM/F12 supplemented with 10% non-heat-inactivated FBS (GIBCO); SUM159T and MCF10A were grown in DMEM/F12 supplemented with 5% FBS, Insulin 5 μg ml −1 (Sigma) and Hydrocortisone 0.5 μg ml −1 . (Sigma). For cell transfection, Lipofectamine-2000 (Invitrogen) was used, according to manufacturer's instructions. Cell viability assay Cell viability was assessed by automated Trypan-Blue exclusion staining (Countess, Invitrogen), according to the manufacturer's instructions. Clonogenic assay Briefly, semiconfluent breast cancer cells were exposed to a short pulse of Metformin (0.5 mM per 3 h), and subsequently seeded at 1,000 cells per well into 6-well dishes (Costar). Number of colonies was scored by Cristal Violet staining 10 days later. NMR sample preparation Extracellular metabolites were separated by ultrafiltration (Amicon). Cell pellets and tissue samples were lyophilized, weighted and cryogenically grounded using Cryomill (Retsch GmbH Germany) before methanol/chloroform/water extraction (2/2/1.8) to extract nonpolar metabolites [44] , [45] . Hydrogen1-nuclear magnetic resonance ( 1 H-NMR) spectroscopy For the Hydrogen-( 1 H) nuclear magnetic resonance ( 1 H-NMR) analysis, polar extracts were dissolved in 600 μl of 1 mM TSP ((trimethylsilyl)-propionic-2,2,3,3-d 4 acid) and 10 mM NaN 3 solution in D 2 O 0.1 M. phosphate buffer (pH=7.4), while nonpolar extracts were dissolved in 600 μl of CDCl 3 containing 0.03% TMS (tetramethylsilane)/CD 3 OD solution (2:1, v/v). All 2D 1 H J-resolved (JRES) NMR spectra were acquired on a 500-MHz DRX Bruker Avance spectrometer (Bruker, Germany), using a double spin-echo sequence with 8 transients per increment for a total of 32 increments. These were collected into 16 k data points using spectral widths of 6 kHz in F2 and 40 Hz in F1. There was a 3.0-s relaxation delay. The water resonance was suppressed using presaturation. Each free induction decay (FID) was Fourier transformed after a multiplication with sine-bell window functions in both dimensions. JRES spectra were tilted by 45°, symmetrized about F1, referenced to TSP at δ H =0.0 p.p.m. and the proton-decoupled skyline projections (p-JRES) exported using Bruker's XWIN-NMR software. Metabolites were identified using an in-house NMR database and literature data and confirmed by 2D homo- and hetero-nuclear NMR spectroscopy. 31 P-NMR spectroscopy For 31 P-NMR analysis nonpolar tissue extracts were recovered after the 1 H-NMR analysis, N 2 -dried and redissolved in a mixture of CDCl 3 /CH 3 OH/0.2 M. aq. K 2 EDTA (pH=6.0) (100:29.9:5.2, v/v/v). 31 P-NMR spectra of nonpolar tissue extracts were obtained at the observation frequency of 202.5 MHz using a standard Bruker single pulse 1H-decoupled experiment with the following parameters: flip- angle of the excitation pulse 60°, acquisition time 0.82 s, relaxation delay 1.0 s, 2,880 transients. Data processing was performed on Lorentz–Gauss transformed spectra with the line broadening of 1.0 Hz. 1,2-diacyl-sn-glycero-3-phosphocholine was used as chemical-shift reference compound (−0.84 p.p.m.). 1 H and 31 P-NMR spectra pre-processing All p-JRES exported were aligned and then reduced into spectral bins with widths ranging from 0.01 to 0.02 p.p.m. by using the ACD intelligent bucketing method (ACD/Labs, Canada) that sets the bucket divisions at local minima (within the spectra) to ensure that each resonance is in the same bin throughout all spectra. After this procedure, the 1 H spectra were divided into n bins. The area within each spectral bin was integrated to yield an n -component vector, where each component value was represented by the integral value corresponding to the specific spectral bin. To compare the spectra, the integrals derived from the bucketing procedure were normalized to the total integral region, following exclusion of bins corresponding to solvent (residual water/HDO, δ 4.76–4.82 p.p.m. ; CDCl 3 , δ 7.45-7.50 p.p.m. ; CD 3 OD, δ 3.33–3.37 p.p.m. ), TSP, TMS (δ−0.5 to 0.5 p.p.m.) and metformin peaks (δ 3.03–3.06 p.p.m.). Data from extracellular media were expressed in terms of net balances at 0 and 24 h. This was done to illustrate the consumption (c) or production (p) of the selected metabolites in time. For cell pellets and tissue samples, the data set was constituted by a matrix having as rows cell or tissue samples and as columns the integral values of polar and nonpolar metabolites determined by 1 H- (for cell pellets and tissue samples) and 31 P-NMR (for tissue samples) spectroscopy. 13 C-NMR spectroscopy For 13 C-NMR analysis, cells were incubated for 24 h in complete medium containing 3 g l −1 [1,2- 13 C2] glucose to obtain an isotopic steady-state labelling, and processed as indicated. Phase-sensitive gradient-enhanced [ 13 C, 1 H] HSQC spectra were acquired on a 700-Mhz DRX Bruker Avance spectrometer, with a TCI cryoprobe (Bruker, Germany) with 4 transient per increment for a total of 2,000 increments. These were collected into 2 k data points using spectral widths of 8 kHz in F2 and 32 kHz in F1. A relaxation delay of 1.5 s was used. The resulting spectra were processed in Bruker's Topspin software using standard methods. Statistical analysis The resulting data was used as input for univariate and multivariate analysis PCA [34] and OPLS-DA [35] . PCA and OPLS-DA were conducted using SIMCA-P+ version 12 (Umetrics, Umea, Sweden). Western blotting The following primary antibodies were used: anti phospho-AMPKα (Thr-172) (Cell Signaling, #2531); anti-phospho-Raptor (Ser-792) (Cell Signaling, #2971); anti-phospho-mTOR(Ser-2448) (Cell Signaling, #2083); anti-beta actin (A-2228, Sigma); anti c-MYC (Santa Cruz, sc-40), anti-DICER (Santa Cruz, sc-30226), anti-HIF1alpha (BD Transduction Laboratories, #610959), anti-IRS2 (Cell Signaling, #3089). All the indicated antibodies were used at the minimum dilutions suggested by the manufacturer. The Image J software was used to quantify the obtained data, according to the manufacturer's instructions. RNA processing and hybridization Total RNA from breast cancer cell lines was extracted by TRI Reagent lysis reagent (Ambion), according to manufacturer's instructions. Agilent's microRNA Complete Labeling and Hyb Kit (Agilent) was used to generate fluorescent microRNA, according to manufacturer's instructions. Scanning and image analysis were performed using the Agilent DNA Microarray Scanner (P/N G2565BA). Feature Extraction Software (V-10.5) was used for data extraction from raw microarray image files using the miRNA_105_Dec-09FE protocol. Statistical analysis For microRNA analysis, Pearson's correlation coefficient was calculated to assess quality of replicates. ANOVA test (α=5%) was performed to assess statistical significance of the observed differences in microRNA profiling ( Supplementary Fig. S2 ). Generally, Student's t -test was used to assess significance of the data whereas the significance of mice survival data was determined by using Kaplan–Meier analysis and Mann–Whitney test ( Fig. 1b ). P -values ≤0.05 were considered statistically significant. MicroRNA analysis The whole bioinformatic analysis was performed by in-house MATLAB scripts. Prediction of the engaged pathways was performed with DIANA software ( http://diana.cslab.ece.ntua.gr ), with manual annotation of the tissue-specific pathways. The microarray data can be accessed at http://www.ncbi.nlm.nih.gov/geo (accession number: GSE37038 ). Hypoxia induction Cells were seeded at 1*106 cells per 60 mm in tissue culture glass dishes and grown for 24 h in complete medium. Medium was changed to serum-free medium and cells incubated in specially designed glass chambers flushed with 5% CO2 and 95% N 2 . After 24 h, cells were collected and immediately processed for further analysis. Wound healing assay Briefly, SUM159PT cells were grown to 80% confluence in 6-well tissue culture plates and wounded with a sterile 10-μl pipette tip to remove cells by two perpendicular linear scrapes. The progression of migration was photographed at the indicated times. Xenograft transplantation studies 4–6 weeks CD1 nude mice (Charles River) were subcutaneously transplanted with SUM159PT cells (1×10 6 cells per mouse) and treated as indicated up to the termination of the study. Tumour volume (cm 3 ) was calculated as follows: 0.5×D 1 2 ×D 2 , where D 1 and D 2 are the larger and smaller diameters measured by caliper. All tumorigenicity assays were carried out according to the guidelines set by the Internal Ethical Committee. Necroscopy was performed for all the mice at the end of the study by expert pathologists, under magnifying glasses. Immunohistochemistry Formalin-fixed, paraffin-embedded sections of mice tumours were stained with Haematoxylin and Eosin or stained with anti-Ki-67 antibody (1:200, Ventana, Roche). Viral infections Briefly, lentiviral vectors coding for DICER-targeting shRNAs were transfected in 293 cells in combination with pMDG and pCMV8.74. to obtain viral particles used to infect SUM159PT cells. Psico-DICER (targeting shRNA) #1-3 were from Addgene (UK) (plasmids 14763-14764-14765) (Kumar, 2007 #1736). psicoR-pGK-puro vector (Addgene plasmid-12084) was used as a control ( Supplementary Fig. S3A ). PLKO.1-shRNA#4 was a gift of Dr. Stefano Piccolo (Padua, Italy). The scrambled-shRNA consisted of an shRNA insert that contains 4 base pair mismatches to any known human or mouse gene in the same backbone vector (PLKO.1) (SIGMA- SHC002). The DICER RNAi-stable vector (pRRL-DICER CDS) was a gift of Dr. Stefano Piccolo. Luciferase assays The full length 3′ UTR of the human c-MYC genes were amplified and inserted downstream of the Renilla luciferase gene into the NotI sites of the dual luciferase reporter plasmid PSICHECK-2 (Promega). For 3′-UTR reporter assays cells were co-transfected in 24-well plates psiCHECK2-cMyc-3′UTR or PSICHECK2 (as a control) together with 40 nM of miR-33a inhibitor or control (miRIDIAN, Thermo Scientific-Dharmacon). After 24 h, cells were treated with vehicle or metformin and extracts analysed using the Dual Luciferase kit (Promega). Cell-cycle analysis For cell-cycle analysis, cells were stained 30 min at room temperature (RT) with propidium iodide (50 μg ml −1 PI, 0.5 mg ml −1 ; RNAse in PBS) before flow-cytometric analysis. qPCR qPCR assays were performed by STEPOne PCR using the FastStart SYBR Green Master Mix (Applied Biosytems). Sequences of qPCR primers are DICER Fw: 5′-CAAGTGTCAGCTGTCAGAACTC-3′, Rv: 5′-CAATCCACCACAATCTCACATG-3′. IRS-2 Fw 5′-ACGCCAGCATTGACTTCTTGT-3′, Rv :5′-GCCAGACAGATCTTCACTCTTTCA-3′ ACTIN Fw: 5′-GGCATGGGTCAGAAGGATT-3′, Rv: 5′-CACACGCAGCTCATTGTAGAAG C-MYC-3′ Fw: 5′-CTCCTGGCAAAAGGTCAGAG-3′, Rv: 5′-TCGGTTGTTGCTGATCTGTC-3′, HIF1α−Fw: 5′-CCCCAGATTCAGGATCAGACA-3′, Rv: 5′-GGACTATTAGGCTCAGGTGAACTTTG-3′. Chromatin immunoprecipitation Pre-cleared chromatin was incubated overnight with the following antibodies: anti-E2F3 (Santa Cruz Biotechnology #251), anti-E2F5 (Santa Cruz Biotechnology, #999), anti acetylH4 (Upstate #06–866), anti p300(N-15) (Santa Cruz Biotechnology, #584), anti-RNA polymerase II CTD(phospho Ser5) (Abcam, #5131), anti-Phospho RNA Polymerase II (phospho ser2) (Bethyl #A300-654A). All the CHIP antibodies were used at 4 micrograms per ml of diluted chromatin. Semiquantitative and quantitative PCR were used to assess for DNA enrichment. Primer sequences used (for E2F binding sites: NM_177438) are E2F3 (DICER)Fw: 5′-TCTGCCAAACTTAGCCGGCCTC-3′, Rv: 5′-GAGCCTGTGATTGGACAGGGCCT-3′; E2F5 (DICER)Fw: 5′-GCGGAAGTGGGTGTTTGTTATT-Rv: 5′-GCGTTTCCTCGCGTTAGTG-3′; cyclin-B1 intron (control) Fw: 5′-GGAGTCTCTATCGGCTCTTATACCG-3′ Rv: 5′-GTCCAGTTTCCCAAGGCCAAT-3′. Accession codes: The microarray data have been deposited in the Gene Expression Omnibus under accession number GSE37038 . How to cite this article: Blandino, G. et al . Metformin elicits anticancer effects through the sequential modulation of DICER and c-MYC. Nat. Commun. 3:865 doi: 10.1038/ncomms1859 (2012).